Large recovery strain in Fe-Mn-Si-based shape memory steels obtained by engineering annealing twin boundaries Shape memory alloys are a unique class of materials that can recover their original shape upon heating after a large deformation. Ti-Ni alloys with a large recovery strain are expensive, while low-cost conventional processed Fe-Mn-Si-based steels suffer from a low recovery strain (<3%). Here we show that the low recovery strain results from interactions between stress-induced martensite and a high density of annealing twin boundaries. Reducing the density of twin boundaries is thus a critical factor for obtaining a large recovery strain in these steels. By significantly suppressing the formation of twin boundaries, we attain a tensile recovery strain of 7.6% in an annealed cast polycrystalline Fe-20.2Mn-5.6Si-8.9Cr-5.0Ni steel (weight%). Further attractiveness of this material lies in its low-cost alloying components and simple synthesis-processing cycle consisting only of casting plus annealing. This enables these steels to be used at a large scale as structural materials with advanced functional properties. Shape memory alloys (SMAs) are fascinating materials that are characterized by a shape memory effect (SME) and superelasticity, which conventional metals and alloys do not have [1] , [2] , [3] . When they are deformed below a certain temperature, they can recover their original shape when heated above a critical temperature, that is, revealing the SME [2] , [3] . When deformed above a critical temperature, they can recover a large nonlinear strain above several percent upon unloading, an effect that is referred to as the superelasticity [2] , [3] . Among the studied SMAs, polycrystalline Ti-Ni-based alloys have found applications in pipe couplings and actuators owing to their excellent SME and superelasticity [3] . Unfortunately, Ti-Ni-based alloys are very expensive owing to their low productivity and the high-cost fabrication caused by the expensive alloy ingredients and their low cold workability [4] . Therefore, low-cost polycrystalline shape memory steels (SMSs), such as Fe-Mn-Si [5] , [6] , [7] , [8] , [9] , [10] , [11] , [12] , [13] , [14] , [15] , Fe-Ni-C [16] and Fe-Ni-Co-Ti [17] , [18] , [19] , have been developed. Recently, a major breakthrough in the superelasticity has been made in the polycrystalline SMSs. Tanaka et al. [4] reported a huge superelastic strain >13% at room temperature in an Fe-28Ni-17Co-11.5Al-2.5Ta-0.05B steel (atom%), and Omori et al. [20] attained a superelasticity of >6% in an Fe-34Mn-15Al-7.5Ni steel (atom%) with a mean grain size of ~3.8 mm and a bamboo structure. Such huge superelastic strains have never been observed before in polycrystalline SMSs. However, so far, a large recovery strain (RS) resulting from the SME has not been reported for the polycrystalline SMSs except for single-crystalline Fe-30Mn-1Si steel showing 9% RS (ref. 5 ) and melt-spun Fe-16Mn-5Cr-6Ni-3Si-0.2B steel thin foil showing 7.2% RS (ref. 21 ). Although it is beyond doubt that the SME in the Fe-Mn-Si-based steels results from the stress-induced transformation of gamma (γ) to epsilon martensite (ε) (abbreviated to SIEM) [3] , [5] , the critical factor in controlling their RS has been under intense discussion. Otsuka et al. [6] and Gu et al. [8] suggested that for obtaining a large RS, the alloying design in the Fe-Mn-Si-based steels should satisfy the following two main criteria: (1) the stacking fault energy (SFE) should be as low as possible to facilitate the SIEM transformation; and (2) the start temperature of the γ to ε transformation, M s , should be just below the deformation temperature so that no thermally induced ε exists before the deformation. However, a recent study by Stanford et al. [11] showed that the SME increased with higher SFE. Wayman and colleagues [7] reported that the pre-existing thermally induced ε did not deteriorate the SME when the deformation was not too large. In addition, some studies showed that irrespective of the chemical composition, the RS of the Fe-Mn-Si-based SMSs can be improved up to ~5% from 2–3% by training, that is, the repetition of a cycle consisting of 3–5% tensile deformation at room temperature and subsequent annealing between 873 and 923 K (refs 6 , 22 , 23 , 24 , 25 , 26 ). In addition to this special thermo-mechanical treatment, both the thermo-mechanical treatment of a tensile deformation at 973 K, that is, ausforming [27] , [28] and that of 10% cold rolling and subsequent annealing at ~973 K can remarkably enhance their RS [9] , which is also independent of the specific chemical composition. Accordingly, the chemical composition is not the critical factor in controlling the RS in the Fe-Mn-Si-based SMSs. Kajiwara et al. [9] , [29] , [30] suggested that to obtain a large RS, the austenite grains must contain a high density of uniformly distributed stacking faults (SFs) based on the detailed microstructural investigations of the SIEM in a trained Fe-14Mn-6Si-9Cr-5Ni steel (weight% here and after), and the role of the training is to introduce this type of SFs. However, the recent study by Stanford et al. [31] showed that although few SFs existed in an Fe-Mn-Si-Cr-Ni steel subjected to hot rolling at 1,373 K and then annealing at 873 K, its RS is comparable to the one observed in the trained state. This result suggests that a high density of pre-existing SFs is also not the critical factor for obtaining a large RS in the Fe-Mn-Si-based SMSs, although their introduction is assumed to provide nucleation sites for the SIEM and is thus favourable for their RS enhancement [9] . The Fe-Mn-Si-based SMSs are face-centred cubic (FCC) metals with very low SFE. For the FCC metals with intermediate or low SFE, a commonly observed feature is the presence of copious parallel-sided annealing twin lamellae after thermo-mechanical processing, usually involving cold working followed by annealing. Especially, these annealing twins are always bounded by {111} planes or coherent twin boundaries (TBs), apart from a few short incoherent steps and terminations [32] . Therefore, a high density of annealing TBs, including dominant coherent TBs and a few incoherent ones, must exist in the conventional thermo-mechanically processed Fe-Mn-Si-based SMSs. On the other hand, the interfacial energy of coherent TB is only ~5% of the energy of an arbitrary high-angle grain boundary (GB) [32] . Consequently, stronger interactions between the annealing TBs and the SIEM inevitably occur during deformation. Surprisingly, up to now this type of interactions has not been discussed in the literature. In this study, we investigate the evolution of the annealing TBs by electron backscatter diffraction (EBSD) and their resulting effect on the RS in a cold-rolled Fe-18.8Mn-5.0Si-8.5Cr-5.0Ni steel (referred to as 19Mn) before and after the above-mentioned different thermo-mechanical treatments. We find that a high density of the annealing TBs exists in the annealed 19Mn steel, and thus the SIEM–TB interactions are frequently observed during deformation. These interactions not only heavily distort the TBs but also significantly inhibit the SIEM process. Because of the distortion of TBs, the original orientation between the twin and the parent grain cannot recover after recovery heating. After the different thermo-mechanical treatments, a common microstructural feature is the low density of the TBs. In addition, independent of the methods of the thermo-mechanical treatments, a clear negative linear relationship exists between the shape recovery rate (SRR) and the density of the TBs. Through significantly suppressing the formation of the TBs in the microstructure, we attain a bending RS of 8.4% and tensile RS as high as 7.6% in a cast and annealed polycrystalline Fe-20.2Mn-5.6Si-8.9Cr-5.0Ni steel with coarse grains of ~1.10 mm (referred to as-cast 20Mn). 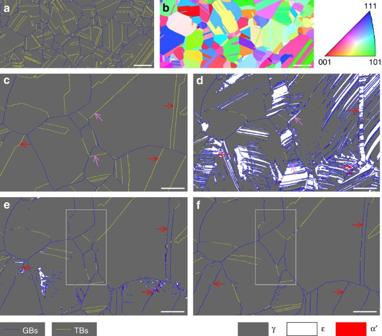Figure 1: Evolution of TBs after deformation and recovery annealing. (a,b) EBSD phase map together with GB character and corresponding inverse pole figure for the cold-rolled 19Mn steel annealed at 1,373 K. Scale bars, 200 μm. EBSD phase maps combining GB character taken on the same surface of a specimen before deformation (c) and after 10% tensile deformation at 293 K (d), and then annealing at 623 K (e) and 773 K (f). Scale bar, 50 μm. Purple arrows show that the stress-induced epsilon martensite nucleates at the TBs; red arrows show that the collisions between the TBs and the stress-induced transformation of gamma (γ) to epsilon martensite (ε) result in an incomplete recovery of original orientation between the twins and the parent grains; white rectangles show the movement of some of the TBs together with the other GBs. EBSD: electron backscatter diffraction; GBs: grain boundaries; TBs: twin boundaries. Evolution of TBs after deformation and recovery annealing Figure 1a,b show EBSD phase maps combining the GB character and the corresponding inverse pole figure for the cold-rolled 19Mn steel annealed at 1,373 K. After annealing, a high density of annealing TBs (yellow lines) exists. The ratio of the total length of the TBs relative to the total length of all GBs including the TBs reaches 56.4%. Figure 1c–f show similar EBSD phase maps taken on the same surface of the 19Mn steel specimen annealed at 1,373 K before and after 10% tensile deformation at 293 K followed by a recovery annealing treatment at 623 and 773 K, respectively. After deformation, some SIEM nucleate at the TBs as indicated by the purple arrows. However, most of the TBs collide with the SIEM in the twins and/or that in the parent grains as indicated by the red arrows. As the result of the collisions, some alpha prime martensite (α′) are produced near the TBs (red particles in Fig. 1d ). Transmission electron microscope (TEM) observations revealed that these SIEM–TB collisions heavily distort the TBs ( Fig. 2 ). After recovery annealing at 623 K, the distorted TBs cannot be identified any more as the TB by the TSL OIM software, although the SIEM revert to the austenite ( Fig. 1e ). In other words, the original orientation between the twins and the parent grains cannot recover after annealing at 623 K. This result indicates that the misorientation across the distorted interfaces must be >65° or <55° because the tolerance of the misorientation relative to the twin is set as 5° in the TSL OIM software. In addition, the introduced α′ cannot revert to the γ ( Fig. 1d,e ). When further annealing, this sample at 773 K, the introduced α′ reverted to austenite, but the original orientation between the twins and the parent grains still cannot recover ( Fig. 1f ). Interestingly, some of the interfaces moved together with the other GBs. This effect becomes evident when comparing the areas designated by the white rectangles indicated in Fig. 1e,f . These unrecovered orientations between the twins and the parent grains mean that the deformed sample shape cannot recover completely. Figure 1: Evolution of TBs after deformation and recovery annealing. ( a , b ) EBSD phase map together with GB character and corresponding inverse pole figure for the cold-rolled 19Mn steel annealed at 1,373 K. Scale bars, 200 μm. EBSD phase maps combining GB character taken on the same surface of a specimen before deformation ( c ) and after 10% tensile deformation at 293 K ( d ), and then annealing at 623 K ( e ) and 773 K ( f ). Scale bar, 50 μm. Purple arrows show that the stress-induced epsilon martensite nucleates at the TBs; red arrows show that the collisions between the TBs and the stress-induced transformation of gamma (γ) to epsilon martensite (ε) result in an incomplete recovery of original orientation between the twins and the parent grains; white rectangles show the movement of some of the TBs together with the other GBs. EBSD: electron backscatter diffraction; GBs: grain boundaries; TBs: twin boundaries. 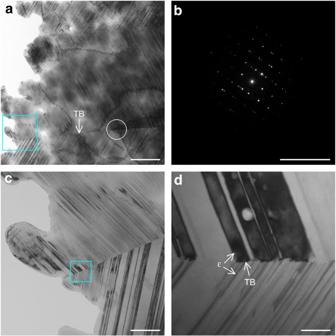Figure 2: Distortion of TB due to interactions between TB and SIEM. (a) Bright-field TEM image for the cold-rolled 19Mn steel annealed at 1,373 K after 10% tensile deformation at 293 K. Scale bar, 5 μm. (b) Selected-area diffraction pattern taken from the white circle area ina, showing that the interface indicated by the white arrow inais the TB. Scale bar, 20 nm−1. (c) Enlarged cyan rectangle area ina. Scale bar, 1 μm. (d) Enlarged cyan rectangle area inc, showing the distortion of the TB. Scale bar, 50 nm. SIEM: stress-induced transformation of gamma (γ) to epsilon martensite (ε); TB: twin boundary. Full size image Figure 2: Distortion of TB due to interactions between TB and SIEM. ( a ) Bright-field TEM image for the cold-rolled 19Mn steel annealed at 1,373 K after 10% tensile deformation at 293 K. Scale bar, 5 μm. ( b ) Selected-area diffraction pattern taken from the white circle area in a , showing that the interface indicated by the white arrow in a is the TB. Scale bar, 20 nm −1 . ( c ) Enlarged cyan rectangle area in a . Scale bar, 1 μm. ( d ) Enlarged cyan rectangle area in c , showing the distortion of the TB. Scale bar, 50 nm. SIEM: stress-induced transformation of gamma (γ) to epsilon martensite (ε); TB: twin boundary. 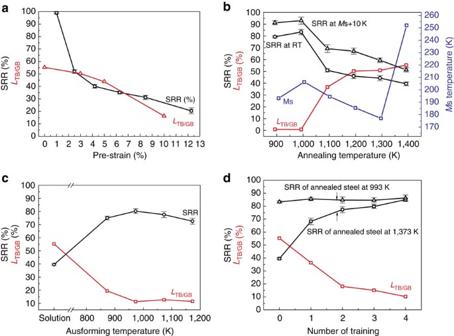Figure 3: Effects of thermo-mechanical treatments on TBs and SRR. (a) Influence of the amount of deformation on the shape recovery rate (SRR) and the ratio of total length of TBs relative to total length of all GBs including TBs (LTB/GB) in the cold-rolled 19Mn steel annealed at 1,373 K. (b) Effects of annealing temperature on theLTB/GB, SRR andMstemperature in the cold-rolled 19Mn steel. (c) Influence of the ausforming temperature on theLTB/GBand SRR in the cold-rolled 19Mn steel annealed at 1,373 K. (d) Effect of the number of training cycles each consisting of 5% tensile deformation at 293 K and subsequent annealing at 923 K for 15 min on theLTB/GBand SRR in the cold-rolled 19Mn steel annealed at 1,373 and 973 K, respectively. Error bars, s.e.m. GBs: grain boundaries;Ms: start temperature of gamma to epsilon martensitic transformation; TBs: twin boundaries. Full size image Effect of thermo-mechanical treatments on TBs and SME Figure 3a shows the effect of bending pre-strain at 293 K on the SRR of the 19Mn steel annealed at 1,373 K. The SRR drops when increasing the pre-strain. Figure 3a also shows the effect of tensile pre-strain at 293 K on the resulting ratio of the total length of the TBs relative to the total length of all GBs including the TBs, L TB/GB . The L TB/GB also drops as the strain increases, showing that the larger the deformation is, the more distorted are the annealing TBs. Figure 3: Effects of thermo-mechanical treatments on TBs and SRR. ( a ) Influence of the amount of deformation on the shape recovery rate (SRR) and the ratio of total length of TBs relative to total length of all GBs including TBs ( L TB/GB ) in the cold-rolled 19Mn steel annealed at 1,373 K. ( b ) Effects of annealing temperature on the L TB/GB , SRR and M s temperature in the cold-rolled 19Mn steel. ( c ) Influence of the ausforming temperature on the L TB/GB and SRR in the cold-rolled 19Mn steel annealed at 1,373 K. ( d ) Effect of the number of training cycles each consisting of 5% tensile deformation at 293 K and subsequent annealing at 923 K for 15 min on the L TB/GB and SRR in the cold-rolled 19Mn steel annealed at 1,373 and 973 K, respectively. Error bars, s.e.m. GBs: grain boundaries; M s : start temperature of gamma to epsilon martensitic transformation; TBs: twin boundaries. Full size image Figure 3b shows the L TB/GB and the M s temperature of the cold-rolled 19Mn steel as a function of the annealing temperature. When the annealing temperature is <993 K, the L TB/GB is only 0.8%, that is, very few annealing TBs exist. However, at >993 K, the L TB/GB rises rapidly and reaches 50.2% at 1,193 K. When the temperature exceeds 1,193 K, the increase of the L TB/GB becomes slower with increasing temperature. The M s point rises with the temperature up to 993 K, above which it drops as a function of temperature up to 1,293 K. However, it rises steeply after annealing at 1,393 K. Figure 3b also shows the effect of the annealing temperature on the SRR when bent by 3.6% at 293 K and slightly above the corresponding M s temperature, that is, at M s +10 K, respectively. The SRR is obviously higher when deformed at M s +10 K than at 293 K. However, regardless of the deformation temperatures, the changes in both SRR values are opposite to the trend observed for the L TB/GB with increasing the annealing temperature, that is, the higher the density of the TBs is, the lower is the SRR. Figure 3c shows the evolution of the L TB/GB in the 19Mn steel annealed at 1,373 K after a tensile deformation by 5% at different high temperatures (ausforming) and the corresponding SRR when bent by 3.6% at 293 K. After ausforming, the increase in the SRR also agrees well with the drop in the density of the annealing TBs. Figure 3d shows the L TB/GB in the 19Mn steel annealed at 1,373 K as a function of the number of training cycles. Each training cycle consists of 5% tensile deformation at 293 K and subsequent annealing at 923 K for 15 min. To compare, the associated SRR when bent by 3.6% at 293 K is shown in Fig. 3d . The training substantially reduces the fraction of the TBs and is accompanied by a remarkable increase in the SRR. After only four training cycles, the L TB/GB drops from 55.3% steeply down to 10.2%, whereas the associated SRR increases from 40 to 85%. Interestingly, the training has little effect on the SRR of the 19Mn steel annealed at 993 K, where only very few TBs occur ( L TB/GB =0.8%), as shown in Fig. 3b . These results directly substantiate that the density of the TBs is indeed the critical microstructural factor in controlling the RS, and reducing the density of the TBs is favourable for the RS improvement. 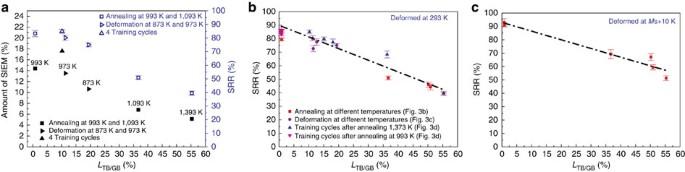Figure 4: Relationship between TBs and SRR. (a) Relationship between the ratio of total length of TBs relative to total length of all GBs including TBs (LTB/GB) and corresponding amount of the SIEM after 4% tensile deformation at 293 K and shape recovery rate (SRR) when bent by 3.6% at 293 K after annealing at different temperatures, ausforming at different temperatures, and four training cycles each consisting of 5% tensile deformation at 293 K and subsequent annealing at 923 K for 15 min for the cold-rolled 19Mn steel. (b) Relationship between theLTB/GBand corresponding SRR when bent by 3.6% at 293 K after different thermo-mechanical treatments for the cold-rolled 19Mn steel. (c) Relationship between theLTB/GBand corresponding SRR when bent by 3.6% atMs+10 K after annealing at different temperatures for the cold-rolled 19Mn steel. Error bars, s.e.m. GBs: grain boundaries;Ms: start temperature of gamma to epsilon martensitic transformation; TBs: twin boundaries. Relationship between density of TBs and SME Figure 4a gives the L TB/GB and the corresponding amount of the SIEM after 4% tensile deformation at 293 K in the cold-rolled 19Mn steel after annealing at different temperatures, ausforming at different temperatures, and four training cycles each consisting of 5% tensile deformation at 293 K and subsequent annealing at 923 K for 15 min. The L TB/GB and the corresponding SRR, when bent by 3.6% at 293 K, are also shown in Fig. 4a . The drop of the L TB/GB agrees well with the increase in the amount of the SIEM and the RS. This means that a high density of the TBs prevents the occurrence of the SIEM, hence deteriorating the SME. Figure 4: Relationship between TBs and SRR. ( a ) Relationship between the ratio of total length of TBs relative to total length of all GBs including TBs ( L TB/GB ) and corresponding amount of the SIEM after 4% tensile deformation at 293 K and shape recovery rate (SRR) when bent by 3.6% at 293 K after annealing at different temperatures, ausforming at different temperatures, and four training cycles each consisting of 5% tensile deformation at 293 K and subsequent annealing at 923 K for 15 min for the cold-rolled 19Mn steel. ( b ) Relationship between the L TB/GB and corresponding SRR when bent by 3.6% at 293 K after different thermo-mechanical treatments for the cold-rolled 19Mn steel. ( c ) Relationship between the L TB/GB and corresponding SRR when bent by 3.6% at M s +10 K after annealing at different temperatures for the cold-rolled 19Mn steel. Error bars, s.e.m. GBs: grain boundaries; M s : start temperature of gamma to epsilon martensitic transformation; TBs: twin boundaries. Full size image Figure 4b gives all L TB/GB and the corresponding SRR when bent by 3.6% at 293 K in the cold-rolled 19Mn steel subjected to annealing at different temperatures ( Fig. 3b ), ausforming at different temperatures ( Fig. 3c ) and different number of training cycles ( Fig. 3d ). Independent of the methods of the thermo-mechanical treatments, a clear negative linear relationship exists between the SRR and the L TB/GB , that is, the lower the density of the TBs is, the higher is the SRR. After annealing at different temperatures, the SRR when bent at M s +10 K also shows a good negative linear relationship with the corresponding L TB/GB ( Fig. 4c ). Thus, it is highly plausible that reducing the density of the TBs is the critical factor for obtaining a large RS in the Fe-Mn-Si-based SMSs. Obviously, identifying simple methods to decrease the density of the TBs is thus a promising direction for developing Fe-Mn-Si-based SMSs with a large RS. Obtaining a giant RS through reducing TBs by simple casting The probability to form annealing TBs is inversely proportional to the SFE [33] . Therefore, increasing the SFE reduces the density of the TBs. This explains the result of Stanford et al. [11] , that is, the RS increases with the rise of the SFE in Fe-29.9Mn-6Si-4.6Cr, Fe-28.4Mn-6Si-6.1Ni and Fe-33.7Mn-6Si steels. Unfortunately, the SFE must be lower than a certain threshold value to make the SIEM take place preferentially [34] . Therefore, reducing the trend to form TBs is limited by adjusting the chemical composition. Fortunately, although a high density of TBs is a characteristic and frequent microstructure feature in the annealed FCC alloys with low SFE, TBs are rarely found in the as-cast alloys. Therefore, we can expect that a larger RS will be obtained in cast Fe-Mn-Si-based SMSs. In fact, recently we attained a high bending RS of 6.4% in a cast and annealed Fe-18Mn-5.5Si-9.5Cr-4Ni steel with lath ferrite [35] . In this paper, we ascribed this result to the grain subdivision effect created by the residual lath ferrite. The analyses given above reveal that the appropriate explanation for the enhanced RS is the low density of TBs in this case. We designed and investigated the RS in cast Fe-Mn-Si-Cr-Ni steels with different Mn contents ( Supplementary Table 1 ). All L TB/GB values in the cast and annealed Fe-Mn-Si-Cr-Ni steels are <10%, that is, only few TBs exist ( Supplementary Table 2 ). Consequently, the RS in the cast and annealed Fe-Mn-Si-Cr-Ni steels is much higher than that of the 19Mn steel annealed at 1,373 K and is comparable to or higher than that of the trained 19Mn steel ( Supplementary Figs 2 and 3 ). Especially, we observe fewer TBs in the cast and annealed 20Mn steel at 1,173 K for 30 min ( Fig. 5a,b and Supplementary Table 2 ) and attain a bending RS of 8.4% ( Fig. 5c , and Supplementary Figs 4 and 5 ) and a tensile RS as high as 7.6% ( Fig. 5d and Supplementary Fig. 6 ). When the tensile pre-strain is <6%, the RS of the cast and annealed 20Mn steel is comparable to that in a single-crystalline Fe-30Mn-1Si steel [5] . More specific, the tensile RS is even larger than that of the well-established Ni-Ti alloys [36] when the pre-strain is >12%, although it is lower when the pre-strain is <12% ( Fig. 5d ). 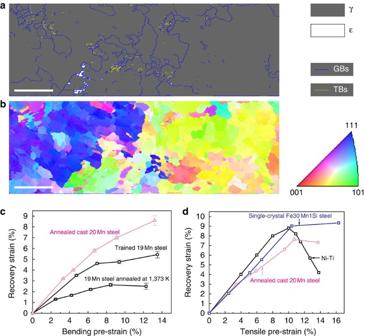Figure 5: Cast and annealed 20Mn steel at 1,173 K showing a giant RS. (a,b) EBSD phase map including the GB character and corresponding inverse pole figure. Scale bars, 1 mm. (c) Effect of bending pre-strain on the RS in the cast and annealed 20Mn steel, the cold-rolled 19Mn steel annealed at 1,373 K and the same material after four training cycles each consisting of 5% tensile deformation at 293 K and subsequent annealing at 923 K for 15 min. Error bars, s.e.m. (d) Effect of tensile pre-strain on the RS of the cast and annealed 20Mn steel, a single-crystalline Fe-30Mn-1Si steel and a polycrystalline Ti-Ni alloy (The RSs of the single-crystalline Fe-30Mn-1Si steel and polycrystalline Ti-Ni alloy were reproduced from the references 5 and 36, respectively). EBSD: electron backscatter diffraction; GBs: grain boundaries; RS: recovery strain; TBs: twin boundaries. Figure 5: Cast and annealed 20Mn steel at 1,173 K showing a giant RS. ( a , b ) EBSD phase map including the GB character and corresponding inverse pole figure. Scale bars, 1 mm. ( c ) Effect of bending pre-strain on the RS in the cast and annealed 20Mn steel, the cold-rolled 19Mn steel annealed at 1,373 K and the same material after four training cycles each consisting of 5% tensile deformation at 293 K and subsequent annealing at 923 K for 15 min. Error bars, s.e.m. ( d ) Effect of tensile pre-strain on the RS of the cast and annealed 20Mn steel, a single-crystalline Fe-30Mn-1Si steel and a polycrystalline Ti-Ni alloy (The RSs of the single-crystalline Fe-30Mn-1Si steel and polycrystalline Ti-Ni alloy were reproduced from the references 5 and 36, respectively). EBSD: electron backscatter diffraction; GBs: grain boundaries; RS: recovery strain; TBs: twin boundaries. Full size image Single-phase solid solution metals without any solid-phase transformation typically form columnar and/or dendritic crystals during solidification. In order to better understand the effect of the associated microstructures and preferred crystallographic orientation obtained in the as-cast state and their influences on the RS, we investigate the effects of specimen size and direction with respect to the solidification direction on the RS ( Fig. 6a,b ). When the tensile pre-strain is <7%, the deviations in the RS of specimens with different thickness and directions are very small. Above 7% pre-strain, the increase in the thickness obviously leads to a drop in the RS. 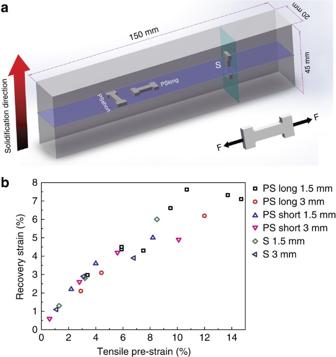Figure 6: Effects of specimen size and direction on RS. (a) Schematic diagram showing the specimen direction with respect to the solidification direction. (b) Effects of the tensile pre-strain on the RS of specimens with different thickness and directions in the cast and annealed 20Mn steel at 1,173 K. RS: recovery strain; PS: perpendicular to solidification direction; S: parallel to solidification direction. Figure 6: Effects of specimen size and direction on RS. ( a ) Schematic diagram showing the specimen direction with respect to the solidification direction. ( b ) Effects of the tensile pre-strain on the RS of specimens with different thickness and directions in the cast and annealed 20Mn steel at 1,173 K. RS: recovery strain; PS: perpendicular to solidification direction; S: parallel to solidification direction. Full size image The giant tensile RS observed in the cast and annealed 20Mn steel, as high as 7.6%, is very surprising and cannot be explained in terms of the low density of TBs alone. In addition, we found that the average grain size in the as-cast 20Mn steel is ~1.10 mm, which is ~8 times that of the cold-rolled 19Mn steel annealed at 1,373 K (including the annealing TBs). Therefore, it is important to clarify whether the grain size or the density of TBs is the critical factor for obtaining a large RS. Effect of TBs intrusion on RS in a coarse-grained cast steel For obtaining coarse grains containing a high density of annealing TBs, we annealed the cast 19Mn steel at 1,373 K for 12.5 h. The L TB/GB increases from 9.2% after 30 min to 25.1% after 12.5 h annealing ( Fig. 7a,b ). After four training cycles, each consisting of 5% tensile deformation at 293 K and subsequent annealing at 923 K for 15 min, the L TB/GB significantly reduces back to 11.7% ( Fig. 7c ). We observe that although the reduction in grain size from ~596 to 499 μm is not substantial owing to the increase in the density of the TBs, however, the drop of the maximal RS value of 6.8% down to only 4.3% is remarkable ( Fig. 7d ). This result directly shows that the increase in the density of the TBs seriously deteriorates the RS. After training, the RS is again increased to 7.4%. This value, however, is only 0.6% higher than that of the sample that was annealed for 30 min. This result again reveals that the introduction of the SFs by training is beyond doubt favourable for improving the RS, but their pre-existence is not a critical factor in controlling the RS. Instead, the low density of the TBs seems to be the dominating critical factor. 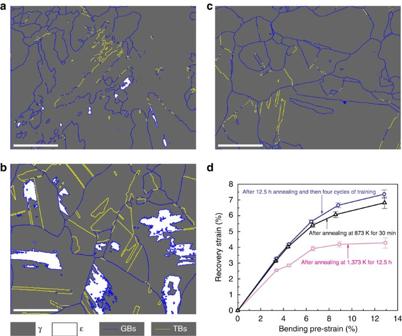Figure 7: Effect of TBs intrusion on RS in a coarse-grained cast steel. EBSD phase maps including the GB character after annealing at 873 K for 30 min (a) and at 1,373 K for 12.5 h (b), and then subjected to four training cycles each consisting of 5% tensile deformation at 293 K and annealing at 923 K for 15 min (c) for cast 19 Mn steel. Scale bars, 500 μm (a–c). (d) Effect of bending pre-strain on the RS after the above mentioned annealing and training. Error bars, s.e.m. TBs: twin boundaries; RS: recovery strain; EBSD: electron backscatter diffraction; GBs: grain boundaries. Figure 7: Effect of TBs intrusion on RS in a coarse-grained cast steel. EBSD phase maps including the GB character after annealing at 873 K for 30 min ( a ) and at 1,373 K for 12.5 h ( b ), and then subjected to four training cycles each consisting of 5% tensile deformation at 293 K and annealing at 923 K for 15 min ( c ) for cast 19 Mn steel. Scale bars, 500 μm ( a – c ). ( d ) Effect of bending pre-strain on the RS after the above mentioned annealing and training. Error bars, s.e.m. TBs: twin boundaries; RS: recovery strain; EBSD: electron backscatter diffraction; GBs: grain boundaries. Full size image The results of Randle et al. [37] revealed that the TBs, especially the coherent TBs, are more effective barriers against plastic flow compared to the GBs in a copper of 99.99% purity because of their lower energy and higher mechanical stability. Also, recent studies show that nanoscale coherent TBs can substantially strengthen the ultrafine-grained metals while preserving acceptable levels of ductility [38] , [39] . Similarly, it can be expected that the TBs, especially the coherent TBs, prevent the onset of the SIEM more efficiently than the GBs do, considering the same requirement of compatible deformation. The present results confirm this. The higher the fraction of the TBs is, the lower is the volume transformed by the SIEM ( Fig. 4a ). Interestingly, the effectiveness of the TBs as obstacles against the SIEM becomes weaker when they are not the TBs any more after the corresponding thermo-mechanical treatments ( Figs 3 and 4 ). The reason may be that the interface energy rises significantly after they lose the twin misorientation, a microstructural configuration with lower energy. As a result, they become more mobile compared to the TBs, and thus they can easily accommodate the interactions between them and the SIEM. This explains that the drop in the density of the TBs is accompanied by the increase in the amount of the SIEM ( Fig. 4a ). The present results show that the annealing TBs also prevent the formation of thermally induced ε martensite. The substantial rise in the fraction of the TBs markedly lowers the M s temperature in the 19Mn steel when annealed between 993 and 1,293 K ( Fig. 3b ). The remarkable grain growth can account for the steep rise of the M s temperature after an annealing treatment at 1,393 K, where the fraction of the annealing TBs is slightly higher when compared to a heat treatment at 1,293 K. For our present cast Fe-Mn-Si-Cr-Ni steels, the solidification mode is ferrite and ferrite-austenite, that is, they solidify primarily as delta ferrite [40] . After the solidification, the delta ferrite transforms into austenite when cooling. This solid state transformation completely destroys the primary delta dendrites, and the resulting GBs and crystallographic orientations are randomized, as shown in Figs 5 and 7 . Consequently, the resulting preferred crystallographic texture is not very strong with respect to the original solidification direction. This is confirmed by the data shown in Fig. 6b . When the tensile pre-strain is <7%, the difference in the RS is very small among the samples prepared from three different directions with respect to the initial solidification direction. For single-crystalline Fe-Mn-Si steel [41] , [42] , however, the RS in specimens deformed along favourable and unfavourable orientations, namely, <414> and <001>, shows a quite large difference by a factor of five. During the deformation of polycrystalline materials, neighbouring grains must undergo compatible deformation. The degree of this grain constraint effect is influenced by the ratio of grain size versus specimen thickness (gs/t). An increase in the gs/t is equivalent to a relaxation of the grain constraints [20] , [43] , [44] , [45] . Accordingly, the increase in the gs/t is favourable for an enhanced SIEM, promoting larger RS values. In polycrystalline bamboo-type Cu-39.8Zn specimen with a mean grain size of ~3 mm, Wayman and colleagues [43] observed a tensile RS as high as 10.2%. In contrast, only a maximum RS of 4.3% was obtained in the specimen with a mean grain size of ~250 μm [43] . The gs/t of the cast and annealed 20Mn steel specimen is 0.74 (1.10/1.50 mm), and that of the 19Mn steel annealed at 1,373 K is 0.087 (0.13/1.50 mm). Thus, the coarse grained state of the cast 20Mn steel sample is assumed to contribute to its giant RS. The average grain size of the cast 20Mn steel is the biggest among the cast steels ( Supplementary Table 2 ), and thus it shows the highest RS value. On the other hand, the degree of the grain constraint effect is more prominent at larger deformation because more independent shear systems must be activated to meet the requirement of compatible deformation. This should be the reason that the increase in the thickness obviously leads to a drop in the RS at larger pre-strain >7% ( Fig. 6b ). In conclusion, we found that a high density of TBs leads to a poor SME in conventional thermo-mechanically processed polycrystalline Fe-Mn-Si-based steels. During deformation, strong interactions take place between the TBs and the SIEM. These interactions not only inhibited the occurrence of the SIEM but also seriously distorted the interfaces of the twins. Consequently, the original orientation between the twins and the parent grains cannot recover after recovery heating. Our results reveal that a clear negative linear relationship exists between the SRR and the density of the TBs, independent of chemical composition, deformation temperature and methods of the thermo-mechanical treatments. Thus, reducing the density of the TBs is the critical factor for obtaining a large RS. Based on this finding, through remarkably suppressing the formation of the TBs, we attained a bending RS of 8.4% and a tensile RS of 7.6% in the cast and annealed Fe-Mn-Si-based steel with fewer TBs. Besides the small density of the TBs, the coarse grained state of the cast steel sample also makes a contribution to its giant RS. Our results provide a fundamental guideline for developing Fe-Mn-Si-based SMSs with a larger RS. Also, we anticipate that understanding the optimal microstructure design of such materials enables further improvement of RS in cast Fe-Mn-Si-based SMSs through modifying and optimizing compositions, solidification and heat treatment parameters. Casting is a versatile and much cost-efficient manufacturing technique, so that our findings will enable wide use of low-cost Fe-Mn-Si-based SMS in many engineering areas as structural materials with advanced functional properties ( Fig. 8 ). 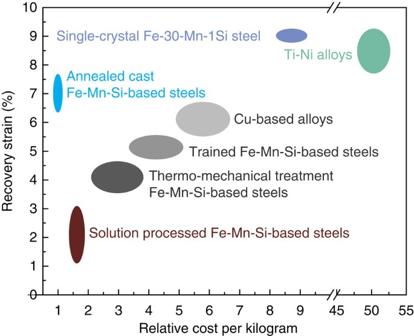Figure 8: Relationship between RS and relative cost per kilogram. RS: recovery strain. Figure 8: Relationship between RS and relative cost per kilogram. RS: recovery strain. Full size image Materials and samples preparation Each ingot of the 'as-cast' Fe-Mn-Si-based steels, 5 kg in weight, was melted and cast into a mould of sodium silicate sand under argon atmosphere in an induction furnace, as shown in Supplementary Fig. 1 . Their chemical compositions are listed in Supplementary Table 1 . For measuring the SME by a bending test, specimens with dimension of 150 × 2.0 × 1.5 mm 3 were cut from the 150 × 20 × 45 mm 3 block of the ingot using a Mo filament cutter. Then they were annealed at different temperatures for 30 min followed by air-cooling. For measuring the SME by an extension test, dog-bone tensile deformation specimens with a gage length of 9 mm, a width of 3 mm and a thickness of 1.5 or 3 mm were cut along different directions with respect to solidification direction, as shown in Fig. 6a . For obtaining sufficient material to produce cold-rolled 19Mn steel, a 15-kg cylinder ingot was cast into a metal mould. After being homogenized at 1,373 K for 15 h, this ingot was hot-rolled into sheets 2.3 mm in thickness at 1,373 K and then solution treated at 1,373 K for 40 min. Finally, they were cold-rolled applying a thickness reduction of ~10% at room temperature. Some of the cold-rolled 19Mn sheets were annealed at different temperatures for 30 min, followed by air-cooling. For performing the training treatment and the ausforming, dog-bone specimens with a gage dimension of 70 × 5 × 2.1 mm 3 were first cut from the cold-rolled 19Mn steel sheets annealed at 1,373 K. Then, some of them were subjected to the training cycles each consisting of 5% tensile deformation at 293 K and subsequent annealing at 923 K for 15 min. The others were tensile-deformed by 5% at different high temperatures, referred to as ausforming. For measuring the SME, specimens with dimension of 70 × 2.1 × 1.5 mm 3 were cut from the annealed sheets, the trained dog-bone specimens and the ausformed dog-bone specimens. The transformation temperatures were determined from the resistivity–temperature curves. Measurements of SME The SME was measured by bending and extension tests. For the bending test, the specimen was bent around a mould with different radii to 180° at 293 K or at M s +10 K for applying a specific amount of pre-strain to the specimen. The pre-strain ε was taken as the maximum tensile strain at the outer edge of the sample thickness, and is determined by the equation: ε = t /(2 R + t ), where R is the bend radius and t is the sample thickness [11] . The bent samples were photographed and then recovery annealed at 773 K for 15 min for shape recovery. After recovery annealing, the residual strain ε r was measured and used to calculate the SRR=100 × ( ε − ε r )/ ε . For the extension test, two indentations were given on the surface of each dog-bone specimen using a Vickers hardness tester. The distance between the two indentations, l 0 , was precisely measured using OLYMPUS CK40M type optical microscope. The marked specimens were tensile-deformed by different amounts at 293 K, and then the distance between the two indentations on each specimen, l 1 , was again measured accurately. Finally, the deformed specimens were recovery annealed at 773 K for 15 min for shape recovery, and then the distance between the two indentations on each specimen, l 2 , was measured accurately. The SRR was calculated by the equation: SRR=100 × ( l 1 − l 2 )/( l 1 − l 0 ). Microstructural characterization The amount of SIEM was determined by XRD using an X′ Pert Pro MPD X-ray diffraction apparatus. The details of the different microstructures were observed by TEM using a Philips CM20 transmission electron microscope. The GB character distribution was determined by using a 6500F JEOL field-emission gun-scanning electron microscope equipped with a TSL OIM EBSD system at 15 kV acceleration voltages. The tolerance of twin misorientation was set as 5°. A step size of 2 and 10 μm was used to scan the samples of the 19Mn steel and the cast steels, respectively. A step size of 0.2 μm was used to characterize the evolution of phases and the TBs on the same surface of 19Mn steel sample annealed at 1,373 K before and after deformation followed by recovery annealing at 623 and 773 K, respectively. How to cite this article: Wen, Y. H. et al. Large recovery strain in Fe-Mn-Si-based shape memory steels obtained by engineering annealing twin boundaries. Nat. Commun. 5:4964 doi: 10.1038/ncomms5964 (2014).